Multicolour nonlinearly bound chirped dissipative solitons The dissipative soliton regime is one of the most advanced ways to generate high-energy femtosecond pulses in mode-locked lasers. On the other hand, the stimulated Raman scattering in a fibre laser may convert the excess energy out of the coherent dissipative soliton to a noisy Raman pulse, thus limiting its energy. Here we demonstrate that intracavity feedback provided by re-injection of a Raman pulse into the laser cavity leads to formation of a coherent Raman dissipative soliton. Together, a dissipative soliton and a Raman dissipative soliton (of the first and second orders) form a two (three)-colour stable complex with higher total energy and broader spectrum than those of the dissipative soliton alone. Numerous applications can benefit from this approach, including frequency comb spectroscopy, transmission lines, seeding femtosecond parametric amplifiers, enhancement cavities and multiphoton fluorescence microscopy. The term ‘dissipative soliton’ (DS) describes stable, localized structures emerging in nonlinear dissipative systems far from thermodynamic equilibrium (see ref. 1 for a comprehensive review of the DS concept explored in different areas of science). In optics, fundamental properties of DSs such as their stability versus energy, dispersion, nonlinearity, noise and so on [1] , [2] , [3] , [4] are studied together with their temporal and spectral shapes [5] , [6] , interaction with other solitons and formation of multisoliton complexes [7] , [8] . Among others, the DS approach is a powerful technique to generate femtosecond pulses beyond the nJ-level in mode-locked laser oscillators based on fibre or other solid-state media [2] , [3] , [4] , [9] , [10] , [11] , [12] , [13] . Broadband, high-energy oscillators can afford numerous applications [14] , [15] , [16] , [17] , [18] . Here we demonstrate a new way of generating broadband complexes in DS oscillators by using nonlinear effects, in our case stimulated Raman scattering (SRS). SRS is observed in an all-fibre (30-m long) 20-nJ DS laser as a limiting effect converting the DS energy to a noisy Stokes-shifted Raman pulse (RP) [9] , which may also lead to DS destabilizations [10] . In ref. 11 , we showed both theoretically and experimentally that in the absence of strong filtering, the SRS effect does not destroy DS preventing, however, further DS energy growth. The noisy RP can even stabilize the DS by means of a nonlinear temporal-spectral filtering [11] resulting in DSs generated in up to 120-m laser cavities. Here we report on a fundamental step forward demonstrating a coherent multicolour complex of bound chirped DSs, one or two of which are the Raman DSs (RDS) generated by SRS process. Numerical simulation In refs 9 , 11 , the noisy RP was observed in the scheme shown in Fig. 1 excluding the Raman feedback loop. The RP evolution in a cavity without feedback is shown in the left column of the diagrams in Fig. 1 . The RP noise is ascribed to the fact that it starts from spontaneous emission reaching high energy after only one round trip of the DS that acts as a pump for the RP. Because of the difference in group velocities, the RP afterwards runs away from the DS. 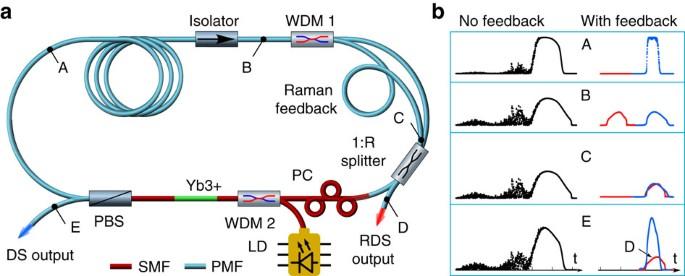Figure 1: Schematic of the laser and calculated pulse shapes. (a) A short (2 m) conventional SMF part providing overdriving-free nonlinear-polarization-evolution (NPE) mode-locking and pulse amplification, and a long (40 m) polarization-maintaining fibre (PMF) part providing dissipative soliton (DS) formation. The Raman feedback loop provides dispersion-compensating delay for the RP directed into the bypass fibre by a wavelength-division multiplexer (WDM1) and its re-injection into the cavity (with coefficient R) via 1:R fibre splitter with output port D. The bypass piece of fibre between WDM1 and 1:R splitter for RP is 12 mm longer than the corresponding piece for DS. The active Yb3+-doped fibre is pumped by a laser diode via the WDM2 coupler. The polarization is controlled by a polarization controller (PC) and is split into orthogonal components by a polarization beam splitter (PBS) with the output port E. (b) The calculated shapes of the generated pulses in the corresponding points (A, B, C, D and E) of the laser scheme, without feedback and with feedback for the Stokes-shifted Raman pulse (RP). Figure 1: Schematic of the laser and calculated pulse shapes. ( a ) A short (2 m) conventional SMF part providing overdriving-free nonlinear-polarization-evolution (NPE) mode-locking and pulse amplification, and a long (40 m) polarization-maintaining fibre (PMF) part providing dissipative soliton (DS) formation. The Raman feedback loop provides dispersion-compensating delay for the RP directed into the bypass fibre by a wavelength-division multiplexer (WDM1) and its re-injection into the cavity (with coefficient R) via 1:R fibre splitter with output port D. The bypass piece of fibre between WDM1 and 1:R splitter for RP is 12 mm longer than the corresponding piece for DS. The active Yb 3+ -doped fibre is pumped by a laser diode via the WDM2 coupler. The polarization is controlled by a polarization controller (PC) and is split into orthogonal components by a polarization beam splitter (PBS) with the output port E. ( b ) The calculated shapes of the generated pulses in the corresponding points (A, B, C, D and E) of the laser scheme, without feedback and with feedback for the Stokes-shifted Raman pulse (RP). Full size image The question arises: what happens if a RP starts not from noise, but from a Raman pre-pulse? If the pre-pulse is re-injected into a laser cavity with the proper timing and amplitude, provided by the Raman feedback loop as shown in Fig. 1 , it will then be synchronously amplified by the DS circulating in the cavity, similarly to synchronous pumping mode-locking technique [19] , [20] . In our case, the mutual intracavity dynamics of DS and RP is important: stationary pulses are formed from the initial noise after several tens of roundtrips in the cavity (see Supplementary Fig. 1 and the corresponding discussion in Supplementary Note 1 ). The difference in the group velocities of DS and RP is compensated by the bypass fibre of the feedback loop providing a necessary delay for the RP. The all-fibre configuration shown in Fig. 1a is based on a conventional ring scheme of a DS fibre laser with normal dispersion [2] , [3] , [4] , with two key differences. The first one consists in the division of the cavity into two functional parts [9] , [11] : a short single-mode fibre (SMF) and a long polarization-maintaining fibre (PMF) providing, respectively, mode-locking and DS formation. The second one is an adjustable feedback loop that re-injects a variable part of the RP back into the laser cavity. To test the effect of the RP feedback on the pulse structure, we first did numerical simulations. The modelling was based on the generalized nonlinear Schrödinger equation (NLSE) [1] , [2] , [3] with the SRS term taken into account in the framework of a scalar model [21] (for details, see the Methods section). The pulse shapes calculated without and with feedback are compared in the diagrams of Fig. 1 . The detailed pulse evolution in these cases is shown in Fig. 2 . A stable noise-free RP was found for the feedback coefficients R=P f /P =10 −2 –10 −6 , where P is the circulating light power with its small re-injected part P f . Details of the feedback optimization can be found in Supplementary Note 1 . 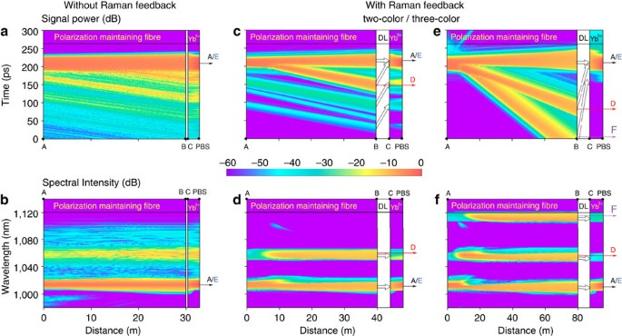Figure 2: Evolution of the pulse shapes and spectra along fibre sections. Shown are PMF and SMF (with the active Yb3+-doped part) sections in a scheme ofFig. 1without feedback (a,b) and with the Raman feedback loop comprising the delay line (DL) shown as the white box, with parameters like in the experiment (c,d). Points A, B, C, D and E, and PBS (polarization beam splitter) of the schemeFig. 1are marked at the corresponding distances. Panelse,fillustrate stable pulse evolution in the case of two feedback loops providing delay and filtering for the first and second Stokes waves with the additional output port F (for details seeSupplementary Note 5). Figure 2: Evolution of the pulse shapes and spectra along fibre sections. Shown are PMF and SMF (with the active Yb 3+ -doped part) sections in a scheme of Fig. 1 without feedback ( a , b ) and with the Raman feedback loop comprising the delay line (DL) shown as the white box, with parameters like in the experiment ( c , d ). Points A, B, C, D and E, and PBS (polarization beam splitter) of the scheme Fig. 1 are marked at the corresponding distances. Panels e , f illustrate stable pulse evolution in the case of two feedback loops providing delay and filtering for the first and second Stokes waves with the additional output port F (for details see Supplementary Note 5 ). Full size image The RP and DS co-propagate together as one stable two-colour complex. For oscillator cavities longer than 80 m, the complex becomes unstable. In the range of cavity lengths supporting the stable complex, increase of the pump power leads to a multipulse regime similar to conventional solitons [7] , [8] , [22] , [23] , [24] . Within each complex, the energy is nearly equally divided between the DS and the noise-free RP (see A and B in Fig. 1b in right column). The pulse evolution along the cavity ( Fig. 2c,d ) demonstrates how a stable noise-free RP is formed at the beginning of PMF due to conversion of the ‘red’ part of the DS into the Stokes-shifted wavelengths ~1,060 nm. Then the DS and RP separate due to dispersion. The delay line in the feedback loop compensates the dispersion shift and after partial outcoupling through ports D and E, and amplifying in Yb 3+ fibre, evolution starts again at point A. As can be seen, the feedback makes pulse evolution basically different (compare Fig. 2c,d with Fig. 2a,b ). The noise is eliminated and the energy becomes concentrated in well-defined temporal and spectral ranges. Other spectral and temporal representations of the noise-free RP are shown in Figs 3 and 4 . Analysis of its spectral and temporal shape together with the spectral phase shown in Fig. 4b led us to the conclusion that the noise-free RP realized numerically in the scheme shown in Fig. 1 can be called a RDS. More details about evolution of the complex involving nonlinear filtering and arguments why our noise-free RP is a chirped DS can be found in Supplementary Note 2 supported by Supplementary Fig. 2 (illustrating the energy fluxes in the complex) and Supplementary Fig. 3 (illustrating variation of the temporal and spectral shapes for DS and RDS, respectively, in six points along the cavity). We also found that the shape of the RDS is very sensitive to parameters of linear spectral filters, just like for conventional DSs (see Supplementary Figs 4 and 5 and Supplementary Note 3 ). 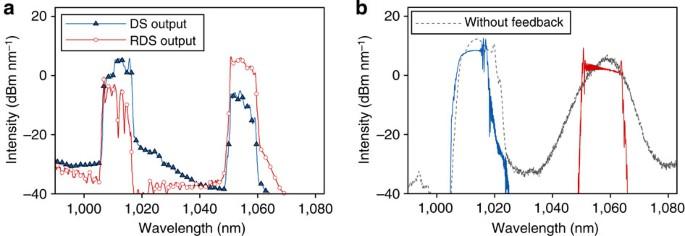Figure 3: Output spectra. (a) Measured and (b) calculated intensity at the DS (blue) and RDS output (red) ports for the 40-m long cavity with the feedback coefficientR=10−4and without feedback (grey). Note that the (i) the spectral division between output ports in the experiment (~10 dB) is not as high as in the simulations (>40 dB); and (ii) the RDS port has significant spectral ripples at ~1,010 nm. Figure 3: Output spectra. ( a ) Measured and ( b ) calculated intensity at the DS (blue) and RDS output (red) ports for the 40-m long cavity with the feedback coefficient R =10 −4 and without feedback (grey). Note that the (i) the spectral division between output ports in the experiment (~10 dB) is not as high as in the simulations (>40 dB); and (ii) the RDS port has significant spectral ripples at ~1,010 nm. 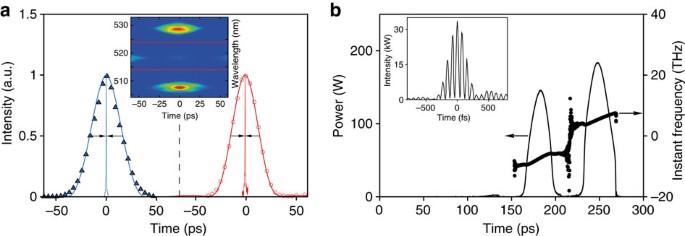Figure 4: Pulse shapes. (a) Points, the measured autocorrelation traces of the DS (blue) and RDS (red), and the calculated (lines) for the 40-m cavity oscillator with the feedback coefficientR=10−4. The dechirped pulses are shown by arrows. Inset: the corresponding FROG traces. (b) The calculated DS and RDS pulse shapes inside the cavity (point B inFig. 1) and their instant frequencies. Inset: the dechirped DS-RDS complex with 70-ps delay in the Raman feedback loop. Full size image Figure 4: Pulse shapes. ( a ) Points, the measured autocorrelation traces of the DS (blue) and RDS (red), and the calculated (lines) for the 40-m cavity oscillator with the feedback coefficient R =10 −4 . The dechirped pulses are shown by arrows. Inset: the corresponding FROG traces. ( b ) The calculated DS and RDS pulse shapes inside the cavity (point B in Fig. 1 ) and their instant frequencies. Inset: the dechirped DS-RDS complex with 70-ps delay in the Raman feedback loop. Full size image In addition to similar characteristics of the RDS and DS: temporal and spectral shapes, chirp and extracavity compression factors, as well as their sensitivity to spectral filtering, the DS nature of the coherent linearly chirped RP was additionally confirmed by its description in the frame of cubic-quintic Ginzburg–Landau equation (CGLE) applicable only for cavities with uniformly distributed parameters. For the sake of comparison of NLSE and CGLE solutions, we made a ‘distribution’ of the point-action terms and solved the CGLE with the average coefficients related to the experimental system (see Methods section and Supplementary Note 4 for details). We compared then the CGLE solutions with the local solutions of the NLSE at the boundary points of the cavity section characterized by uniform evolution of the pulses (points z =12 and 40 m of the PMF; Fig. 2c,d ), and made the arithmetic mean of them supposing that such averaging of the NLSE solutions is comparable with the solution of the CGLE based on the average coefficients. Indeed, one can see in Fig. 5 that the mean NLSE solution for the RDS is very close to the solution of the CGLE with the effective distributed parameters. The CGLE parameters describing the average temporal and spectral shape for the RDS appeared to be close to those for the DS ( Supplementary Note 4 ). In addition, the spectral shape and its chirp are also similar to the measured values presented below. 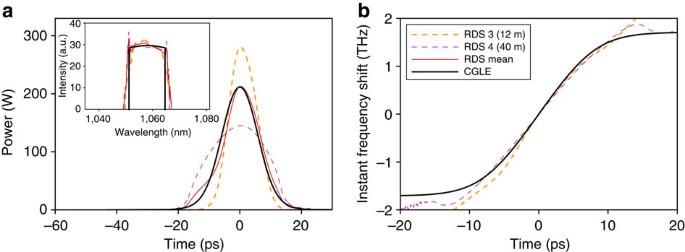Figure 5: Comparison of the NLSE and CGLE solutions. The solutions of CGLE are solid black curves. The pulse parameters are shown for RDS at the cavity pointsz=12 and 40 m of the PMF part (yellow and pink dashed lines, correspondingly) and the arithmetic mean of them (solid red). (a) The pulse power,P=|A|2=|ψ|2/Г, with the corresponding spectra shown in the inset; and (b) the corresponding instant frequency shift (2π)−1dϕ/dtversus timet. Figure 5: Comparison of the NLSE and CGLE solutions. The solutions of CGLE are solid black curves. The pulse parameters are shown for RDS at the cavity points z =12 and 40 m of the PMF part (yellow and pink dashed lines, correspondingly) and the arithmetic mean of them (solid red). ( a ) The pulse power, P =| A | 2 =| ψ | 2 /Г, with the corresponding spectra shown in the inset; and ( b ) the corresponding instant frequency shift (2 π ) −1 dϕ/d t versus time t . Full size image As a next progressive step supporting our concept, we realized a second-order RDS by solving the equation (1); see Fig. 2e,f , and Supplementary Fig. 6 and Supplementary Note 5 for more details). Adding a second feedback loop optimized for the second Stokes wave at 1,110 nm resulted in stable generation of a three-colour DS complex in a 80-m long cavity. Experiment To verify such promising theoretical predictions, we realized experimentally the scheme shown in Fig. 1a (that is, with one feedback loop). The data presented in Figs 3 and 4 showed that the pulses realized in the experiment are basically different from those observed without feedback, but in good agreement with the RDS predicted by simulation. The FROG trace ( Fig. 4 ) shows that the phases, pulse durations and shapes of the DS and RDS are similar. The RDS’s spectrum has a typical shape with steep edges, just like the DS. The duration of the dechirped DS and RDS is measured to be 250–300 fs and 300–400 fs, correspondingly; Fig. 6a,b . The compression factor for the RDS is better than 100, that is, ~30 times higher than that for the noisy RP in refs 9 , 11 , and only slightly lower than that for the DS. The measured interferometric autocorrelation function for the RDS has a contrast close to 8:1 ( Fig. 6a,b ), only slightly deviating from that for the dechirped DS. A radio-frequency beat signals measured at the fundamental repetition rate and its 150th harmonic are also similar for the DS and RDS, exhibiting a high contrast in the range of 60–100 dB ( Fig. 6c,d ). These values are comparable to those for the ~10-nJ SRS-free DS generated in all-fibre configurations of Yb-doped fibre oscillators (for example, ref. 25 ) and only slightly worse than the best results for the ~3-nJ Er-doped fibre oscillators [26] . In our case, the total pulse energy at the DS and RDS outputs is 25 nJ, with nearly equal division inside the cavity and a fourfold difference at the outputs because of selective DS amplification. 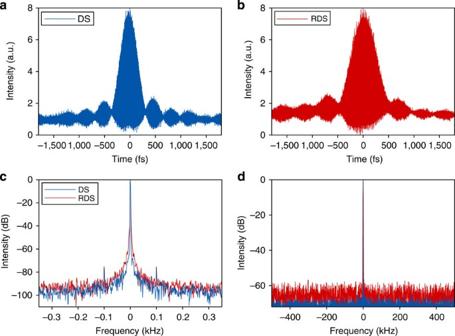Figure 6: Auto-correlation traces and radio-frequency beating spectra of the realized pulses. Traces are shown for DS (a) and RDS (b) after a double-pass compressor consisting of a grating pair. The compressor introduces one-pass group delay dispersion ofD≈−0.7 ps2. Spectra measured at a repetition rate of 5 MHz with 1 Hz bandwidth (c), and at its 150th harmonic (750 MHz) with 1 kHz bandwidth (d). Figure 6: Auto-correlation traces and radio-frequency beating spectra of the realized pulses. Traces are shown for DS ( a ) and RDS ( b ) after a double-pass compressor consisting of a grating pair. The compressor introduces one-pass group delay dispersion of D ≈−0.7 ps 2 . Spectra measured at a repetition rate of 5 MHz with 1 Hz bandwidth ( c ), and at its 150th harmonic (750 MHz) with 1 kHz bandwidth ( d ). Full size image The first-order RDS described above and shown in details in Figs 1 , 2 , 3 , 4 , 5 , 6 (and in Supplementary Figs 1–6 ) substantially differs from a classical Raman soliton, which is a version of fundamental conservative soliton and appears as a result of the Raman frequency shift in the anomalous dispersion range [19] , [20] , for example, in transmission lines [16] . As the RDS is bound with the DS via a nonlinear Raman process, they are also different from one-colour (that is, of the same spectrum) bound solitons or multisoliton complexes based on Kerr nonlinearity [1] , [7] , [8] , [22] , [23] , [24] . In our case ( Fig. 4b ), the DS and RDS form a stable two-wavelength chirped DS complex that could be dechirped into a single pulse under certain conditions. The fringe pattern in Fig. 4b (inset) results from merging of the compressed coherent DS and RDS pulses behind the compressor. The fringe separation (~40 fs) is defined by the whole spectral range of the solitonic DS+RDS complex, whose compressibility can be similar to the cases of nonlinear spectral broadening in fibre [19] or a Raman-active mode-locked laser [27] . It is worth noting that the fringe visibility, which shows the coherence quality, depends on the feedback, with the highest coherence reached for the values 10 −4 < R <10 −2 . The results of simulation also show that the coherence of the RDS and DS is immune to noise variations in a broad range. We presented above all the basic arguments including the solutions of the two main equations in order to formulate unambiguously that the new stable Raman-shifted pulses demonstrated in this paper are DSs. A fair comparison of NLSE and CGLE is a very demanding task, and here we made the first steps in this direction. The approximation of the uniformly distributed cavity relevant for CGLE is rather rough for any laser generating DSs, since typical amplitude variation at point-action dissipative sections (gain, filtering, outcoupling and so on) of the laser cavity amount to about one order of magnitude, while temporal and spectral widths may exhibit much smaller changes; see refs 2 , 3 and citation therein. The same is true for the new DS generated via Raman process, where the amplitude variations are even stronger because of much higher Raman gain and lower feedback coefficient. The pulse widths are also slowly varying here, just like for conventional DS. We call a new soliton centred at 1,060 nm a RDS in order to emphasize its origin leading to quantitative difference of the pulse dynamics from the main DS at similar qualitative behaviour. The average characteristics of the DS and RDS are nearly the same and close to the DS solutions of CGLE. The pulses are nonlinearly bound during the generation process inside the cavity, but can propagate independently outside the laser cavity. Not only SRS, but also other nonlinear processes may be explored for generating broadband multicolour DS complexes. As demonstrated for the femtosecond solid-state lasers [27] , [28] , the combined action of SRS and four-wave mixing allow intracavity spectral broadening similar to the phenomenon of supercontinuum generation in fibres [14] . Successful pulse synthesis based on the total phase and spectrum control was recently demonstrated for several synchronized few-cycle lasers operating in different spectral ranges [29] and for the light-field synthesizer dealing with a coherent supercontinuum from a single few-cycle laser [30] . Based on our approach, intracavity pulse synthesis looks feasible, with an important advantage that it will be intrinsically stable. In conclusion, we have demonstrated a way of generating stable chirped Raman dissipative solitons in the cavity of a DS fibre laser. Together, they form a multicolour complex of bound DSs. As a proof-of-principle step, we showed in detail first-order and in brief second-order Raman solitons. Next-order cloned Stokes and anti-Stokes chirped dissipative Raman solitons also look feasible—their traces are seen in simulation. The fibre laser is a convenient system for embedding Lego-type spectrally and amplitude-varied delay loops in order to enhance its performance. As an extension of laser schemes, bound SRS-driven DSs implemented in periodic transmission lines may result in higher bit rates and better noise suppression than that for conventional Raman-pumped solitons [16] . In addition to the periodic delay loop, either special fibres with properly designed dispersion for the main and frequency-shifted DSs can be used, or the solitons can be kept together by controlling nonlinearities, for example, Kerr nonlinearity [24] . Propagation model Our numerical model uses the NLSE in a scalar form [19] : where A ( z , t ) is the electric field envelope, β 2 and β 3 are the second- and third-order dispersion coefficients at the central frequency ω 0 , γ = n 2 ω 0 /( cA eff ) is the Kerr nonlinearity coefficient with the nonlinear refractive index n 2 and effective fibre cross-section area A eff for the fundamental mode. We neglect such effects as self-steepening and optical shock formation. The response function R ( t )=(1− f R ) δ ( t )+ f R h R ( t ) includes both instantaneous electronic and delayed Raman contributions, where f R represents the fractional contribution of the delayed Raman response to the instantaneous nonlinear polarization. The Raman response function h R ( t ) defines the Raman gain coefficient, whose spectrum is given by . At typical value f R =0.18 (ref. 19 ) and A eff specified for the PMF used, the calculated peak Raman gain (with the Stokes shift Δ λ =45 nm) is nearly equal to the experimental value of g R ≈2.5 W −1 km −1 (ref. 9 ). In our simulations, we use the multiple-vibrational-mode model for the Raman response, described in ref. 21 . The equation was solved by using the symmetrized split-step Fourier-transform method. The simulations are run until the pulse field reaches the steady state after a certain number of cavity roundtrips, taking into consideration the contributions of the point-action WDM1 (sinusoidal) and WDM2 (stepwise, >1,005 nm) transmission spectra (see Supplementary Fig. 4 for details), amplification in Yb 3+ -fibre and the nonlinear polarization-evolution (NPE)-induced intensity modulation described below. The following fibre parameters are used in the simulations: β 2 =22 ps 2 km −1 and β 3 =0.037 ps 3 km −1 , γ =6 W −1 km −1 . An alternative description is based on the generalized Ginzburg–Landau equation that describes distributed along the cavity average characteristics of the solitons (for details, see Supplementary Note 4 ). Amplification model Amplification in the 15-cm-long Yb-doped active fibre including the effect of gain-induced spectral filtering is considered in the frequency domain using the Lorentzian line shape with a bandwidth of 40 nm, a central wavelength of λ 0 ≈1,030 nm, a small-signal gain coefficient of g 0 (λ 0 )≈170 dB m −1 (25 dB total gain). The gain saturation is modelled according to where E is the signal energy given by is the saturation energy, T R = L /cn is the cavity round trip time. The amplifier noise is simulated with complex ‘white’ noise, which is added to the amplitude of the electromagnetic field after its amplification at each round trip. NPE mode-locking Since the SMF part in our scheme is short (2 m) compared with PMF (40 m), the angle of the NPE-induced polarization rotation in SMF is small. So, we can describe the action of the NPE-based modulator in a scalar form by the quibic–quintic term for the pulse amplitude A ( t ) [22] and rewrite the nonlinear modulator transmission ρ , dependent on incident power P = |A| 2 , in the following form: where ρ min =0.05 characterizes the minimal transmission at low powers and ρ max =0.5 is the maximum transmission at critical power P cr =850 W, which corresponds to the experimental data for the PBS splitting ratio in the DS regime. Delay loop The Raman feedback is inserted as follows. The numerical spectral window is divided into two parts. All the spectral components at the wavelengths above 1,030 nm are shifted by 70 ps in the time domain in order to compensate the delay of the DS relative to the RP. The amplitude of the RP is then multiplied by the factor R (the feedback coefficient) provided by commercially available 1% splitters (one or two set in series). The spectral components <1,030 nm are left without any change. The regime of a stable RDS exists within the delay range 50–80 ps (details in Supplementary Note 1 ). Measurements The spectra and shapes of the pulses have been characterized by conventional optical spectrum analyzer (Yokogawa 6370) and FROG (Mesaphotonics) with the extended range up to 100 ps. The FROG data, see inset in Fig. 4a , have been taken from DS and RDS output ports and combined then together. The interferometric autocorrelation measurements of the dechirped DS and RDS pulses were made with the Avesta AA-20DD autocorrelator. Geometrical limits made it difficult to compress both pulses simultaneously, so it was done separately. Radio-frequency beating spectrum of the pulses were measured with an Agilent N9010A spectrum analyzer. How to cite this article: Babin, S. A. et al . Multicolour nonlinearly bound chirped dissipative solitons. Nat. Commun. 5:4653 doi: 10.1038/ncomms5653 (2014).